Niche derived netrin-1 regulates hematopoietic stem cell dormancy via its receptor neogenin-1 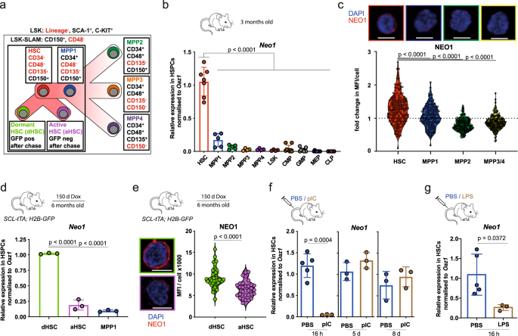Fig. 1: Neo1 is specifically expressed HSC and associated with quiescence. aOverview of hematopoietic stem and progenitor cells (HSPCs) and their immunophenotypes.bRelative expression ofNeo1in HSPCs from 3-month-old mice;n= 4–7 (HSC-MPPs) and 9 (CMP/MEP/GMP), two independent experiments.cMFI of NEO1 in HSPCs from 3-month-old mice;n= 90 (MPP2), 118 (MPP34), 126 (MPP1) and 145 (HSC), two independent experiments.dRelative expression ofNeo1in dHSC and aHSC fromSCL-tTA; H2B-GFPmice, chase for 5 months;n= 3.eMFI of NEO1 in dHSCs and aHSCs fromSCL-tTA; H2B-GFPmice, chase for 5 months;n= 30 (aHSC)–47 (dHSC).fRelative expression ofNeo1in HSCs, 16 h, 5 and 7 days after PBS or poly-I:C injections;n= 3–5 (PBS16h).gRelative expression ofNeo1in HSCs, 16 h after PBS or LPS injections;n= 3 (LPS)–5 (PBS). For all panels, ±SD is shown.nindicates biological replicates. Scale bars in IF images are 5 μm.Pvalue was determined by two-tailedttest. Source data are provided as a Source Data file. Haematopoietic stem cells (HSCs) are characterized by their self-renewal potential associated to dormancy. Here we identify the cell surface receptor neogenin-1 as specifically expressed in dormant HSCs. Loss of neogenin-1 initially leads to increased HSC expansion but subsequently to loss of self-renewal and premature exhaustion in vivo. Its ligand netrin-1 induces Egr1 expression and maintains quiescence and function of cultured HSCs in a Neo1 dependent manner. Produced by arteriolar endothelial and periarteriolar stromal cells, conditional netrin-1 deletion in the bone marrow niche reduces HSC numbers, quiescence and self-renewal, while overexpression increases quiescence in vivo. Ageing associated bone marrow remodelling leads to the decline of netrin-1 expression in niches and a compensatory but reversible upregulation of neogenin-1 on HSCs. Our study suggests that niche produced netrin-1 preserves HSC quiescence and self-renewal via neogenin-1 function. Decline of netrin-1 production during ageing leads to the gradual decrease of Neo1 mediated HSC self-renewal. Haematopoietic stem cells (HSCs) are highly quiescent and give rise to cycling multipotent progenitors (MPPs), which are in turn responsible for maintaining steady-state hematopoiesis [1] , [2] , [3] , [4] , [5] . Upon transplantation, HSCs harbour multilineage and serial long-term engraftment potential [6] , [7] , [8] , [9] . The CD34 − HSC compartment is heterogeneous and consists of both dormant HSCs (dHSCs) and active HSCs (aHSCs) with dHSCs showing superior serial engraftment potential [10] , [11] . dHSCs can be identified via label retention approaches [10] , [11] , [12] , [13] or by employing Gprc5c-GFP reporter mice [11] . All dHSCs reside in a transcriptionally and metabolically rather inactive state and rest in the G 0 cell cycle phase. Upon ageing the number of immunophenotypic HSCs increases, but their self-renewal capability diminishes and a myeloid differentiation bias emerges [14] , [15] , [16] , [17] , [18] , [19] . Various HSC intrinsic hallmarks of ageing, such as the disruption of cellular polarity, and epigenetic instability have been identified [20] , [21] , [22] . Concomitantly, it has become clear that the bone marrow (BM) microenvironment undergoes remodelling upon ageing and contributes to functional decline of HSCs [23] , [24] , [25] . Still, the crosstalk between extrinsic niche-derived and HSC intrinsic factors mediating stem cell maintenance and quiescence, particularly in the context of ageing, remains elusive [26] , [27] . Based on this, we hypothesize that changes in interactions maintaining quiescence in young BM may contribute to the functional decline of HSCs. A number of cell surface receptors, activated by niche-derived ligands such as THPO-MPL, DARC-CD82, or Histamine-H2R, have been described to directly modulate HSC behaviour [28] , [29] , [30] , [31] . Interestingly, some of these, including CXCR4-CXCL12 (C-X-C chemokine receptor type 4/C-X-C motif chemokine 12) and SCF-c-Kit (stem cell factor/c-Kit), also seems to play a key role during neural development [32] , [33] . Neogenin-1 (Neo1), a cell surface receptor first identified as a regulator of axon guidance, has been implicated in a wide variety of functions ranging from cell migration and survival to angiogenesis [34] . Its role has recently also been studied in the innate and adaptive immune systems [35] , [36] , [37] . It shares almost 50% amino acid homology with DCC (deleted in colorectal cancer) [38] , [39] . The extracellular domain of Neo1 has been described to bind members of both the “repulsive guidance molecule” (RGM-a–c) and netrin (Ntn) families [34] , [39] . Neo1 can modulate cytoskeletal activities and can function as a co-receptor for bone morphogenetic proteins (BMPs) [40] , [41] . However, the functional role of Neo1 or its ligands such as Ntn1 in HSC biology remains uncertain [1] , [42] . Here, we identify Ntn1–Neo1 signalling as an important regulator of HSC quiescence. Neo1 is specifically expressed in the most quiescent HSCs Neo1 expression in HSCs has previously been reported by us and others [1] , [42] , [43] , [44] . To further characterize Neo1 expression within the hematopoietic stem and progenitor cell (HSPC) compartment, we isolated various HSPC populations (Fig. 1a and Figure S 1a ) and found Neo1 to be exclusively expressed in HSCs (Fig. 1b ). This HSC-specific expression pattern of NEO1 was also apparent at the protein level (Fig. 1c and Figure S 1b ). NEO1 levels in HSCs were heterogeneous as ~20% of HSCs expressed particularly high levels on the surface (Fig. 1c ). Next, we studied whether this subset of NEO1 high-expressing HSCs corresponds to HSCs (dHSCs) by conducting label-retaining assays using SCL-tTA;H2B-GFP mice [10] (Figure S1c ). After 150 days of doxycycline chase, we found Neo1 transcripts and protein to be expressed at higher levels in dHSCs compared to aHSCs and MPP1s, suggesting that Neo1 is associated with dormancy (Fig. 1d, e ). As expected, dHSCs specifically expressed the dHSC marker Gprc5c [11] (Figure S1d ). To independently validate increased Neo1 expression in dHSCs, we employed Gprc5c-GFP reporter mice and isolated dormant GFP pos and active GFP neg HSCs (Figure S1e ). In agreement, we found higher Neo1 RNA and protein levels in Gprc5c-GFP pos vs. Gprc5c-GFP neg HSCs (Figure S1f, g ). As HSCs are a highly quiescent population during steady state, we next addressed whether Neo1 levels not only rapidly diminished during hematopoietic differentiation, but also upon HSC activation. Therefore, we treated mice with either poly-I:C (pIC) mimicking viral, or lipopolysaccharide (LPS) mimicking bacterial infection [45] , [46] . HSCs showed a robust, reversible loss of Neo1 expression in response to either stimulus (Fig. 1f, g ). Collectively, these data strongly link Neo1 expression to dormancy in HSCs. Fig. 1: Neo1 is specifically expressed HSC and associated with quiescence. a Overview of hematopoietic stem and progenitor cells (HSPCs) and their immunophenotypes. b Relative expression of Neo1 in HSPCs from 3-month-old mice; n = 4–7 (HSC-MPPs) and 9 (CMP/MEP/GMP), two independent experiments. c MFI of NEO1 in HSPCs from 3-month-old mice; n = 90 (MPP2), 118 (MPP34), 126 (MPP1) and 145 (HSC), two independent experiments. d Relative expression of Neo1 in dHSC and aHSC from SCL-tTA; H2B-GFP mice, chase for 5 months; n = 3. e MFI of NEO1 in dHSCs and aHSCs from SCL-tTA; H2B-GFP mice, chase for 5 months; n = 30 (aHSC)–47 (dHSC). f Relative expression of Neo1 in HSCs, 16 h, 5 and 7 days after PBS or poly-I:C injections; n = 3–5 (PBS16h). g Relative expression of Neo1 in HSCs, 16 h after PBS or LPS injections; n = 3 (LPS)–5 (PBS). For all panels, ±SD is shown. n indicates biological replicates. Scale bars in IF images are 5 μm. P value was determined by two-tailed t test. Source data are provided as a Source Data file. Full size image Neo1 -mutant mice reveal a competitive advantage upon transplantation Considering the HSC-specific expression pattern of Neo1 , we set out to study the function of Neo1 in the hematopoietic system. Unfortunately, in our hands, no commercial antibody allowed the robust and reproducible isolation of viable Neo1 + cells by flow cytometry when using Neo1 -mutant cells as controls [42] . Thus, we employed a Neo1 gene-trapped mouse model to genetically address the functional role of Neo1 in HSC biology ( Neo1 gt/gt ) [38] , [47] , [48] . Although Neo1 expression in the BM of mutant mice was diminished by >90% (Fig. 2a ), the hematopoietic compartment did not exhibit altered HSPC or mature cell frequencies in 5–6-week-old animals (Figure S1h ). To analyse Neo1 -deficient hematopoiesis, we performed reconstitution analysis with BM cells derived from 5- to 6-week-old Neo1 -mutant animals (Fig. 2b ). First, we non-competitively transplanted total BM derived from Neo1 -mutant or control littermates (CD45.2) into CD45.1 recipients and assessed HSC numbers 4 months after primary or secondary transplantation (Fig. 2c ). We observed that the frequency of HSCs, while similar at 4 months after transplantation, increased in Neo1 -mutant chimeras upon secondary transplantation. To further investigate this expansion of HSCs, we performed competitive transplantations of Neo1 -mutant or control BM cells (Fig. 2d ). We found that Neo1 -mutant BM cells showed a competitive advantage compared to control counterparts as evident by peripheral blood leucocyte contribution in secondary recipients and in BM HSC contribution in primary and secondary transplantations (Fig. 2e, f ). As HSC frequencies in both transplantation assays increased over time, we also investigated primary chimeras 8 months after transplantation and again found an increase in HSC numbers in Neo1 -mutant chimeras (Fig. 2g, h ). We observed no difference in HSC homing (Fig. 2i, j ), suggesting that self-renewal and output of Neo1 -mutant HSCs are altered. Fig. 2: Mutant Neo1 causes an initial HSC expansion. a Relative expression of Neo1 in the total bone marrow of Wt and Neo1 gt/gt mice; n = 6, three independent experiments. b Workflow: generation of full chimeras. c Absolute frequencies of bone marrow CD45.2 + HSCs in full Wt and Neo1 gt/gt chimeras 4 months after first and second transplantation; n = 5 (2nd Tx)–8 (Ctrl 1st Tx) and 9 (Neo1 1st TX), two independent experiments. d Workflow: competitive transplantations. e Peripheral blood CD45.2 + chimerism during 1° and 2° competitive transplantations of Wt and Neo1 gt/gt bone marrow; n = 13–17 (for exact n /timepoint please see Source data file), three independent experiments, Analysis with two-way ANOVA, multiple comparison with LSD Fisher’s test. f CD45.2 + chimerism of HSCs at endpoints of 1° and 2° competitive transplantations of Wt and Neo1 gt//gt bone marrow; n = 11 (2nd TX), 12 (Ctrl 1st Tx), 14(Neo1 1st TX), three independent experiments. Whiskers are min–max, box is 25–75th percentile and line is mean. g Workflow: full chimeras studied in ( h ). h Absolute frequencies of bone marrow CD45.2 + HSCs in full Wt and Neo1 gt//gt chimeras after 8 months; n = 8 (Ctrl)–9 (Neo1), three independent experiments. i Workflow: Homing assay in ( j ). j Absolute frequencies of CD45.2 + bone marrow LSK cells 48 h after transplantation of 10,000 sorted Wt and Neo1 gt//gt LSK; n = 5 (Ctrl)–6 (Neo1). For all panels, ±SD is shown. n indicates biological replicates. P value was determined by two-tailed t test unless stated otherwise. Source data are provided as a Source Data file. Full size image Aged Neo1 -mutant HSCs display features of premature exhaustion Next, we addressed whether the HSC expansion observed in Neo1 -mutant chimeras would lead to malignant transformation or HSC exhaustion over time (Fig. 3a ). Interestingly, 15 months after the generation of primary chimeras, the initial expansion of the Neo1 -mutant HSC pool reverted and both HSC and MPP1 frequencies decreased (Fig. 3b ). When we compared absolute blood counts in aged Neo1 -mutant chimeras to controls, we found reduced absolute lymphocyte and neutrophil counts, as well as reduced haemoglobin levels indicative of hematopoietic malfunction (Fig. 3c ). As expected, chimeras displayed increased myeloid differentiation upon ageing, and this effect was exacerbated in Neo1 -mutant chimeras over time (Fig. 3d ). To address whether this decline in mature cell output was caused by an HSC defect, we re-transplanted 100 CD45.2 + HSCs derived from either aged Neo1 -mutant or control chimeras (Fig. 3e ). Four months after transplantation, Neo1 -mutant HSCs had generated significantly less progeny then controls (Fig. 3f ). To validate functional exhaustion, we re-transplanted BM of aged chimeras into secondary and tertiary recipients (Fig. 3g ). In these mice, aged Neo1 -mutant BM exhibited a pronounced failure to engraft and depletion of HSCs and all MPP populations was observed, suggesting that the original Neo1 -mutant HSCs from the aged chimeras had a decreased self-renewal potential (Fig. 3h, i ). Meanwhile, we observed no increase in malignancies arising in Neo1 -mutant chimeras. Next, we analysed cell cycle behaviour of Neo1 -mutant HSCs. We found less HSCs residing in the G0 phase in 4–5-week-old Neo1 -mutant mice compared to their control littermates (Figure S1i ). This decrease in G0-HSCs was also apparent in full chimeras both 4 and 8 months after transplantation (Fig. 3j, k and Figure S 1j ) and Neo1 -mutant HSCs expressed higher levels of the cell cycle activation marker CDK6. In addition, increased incorporation of bromodeoxyuridine (BrdU) above the expected injection-induced activation was observed in Neo1 -mutant HSCs (Fig. 3l, m and Figure S 1k ). Altogether, Neo1 -mutant HSCs harbour diminished long-term repopulation potential, associated with a loss of quiescence and increased proliferation. Fig. 3: Mutant Neo1 causes premature HSC exhaustion. a Workflow: aged chimeras, analysed in ( b – d ). b Absolute frequencies of bone marrow CD45.2 + HSPCs in full Wt and Neo1 gt//gt chimeras after 15 months; n = 7 (Ctrl)–11 (Neo1), two independent experiments. c Absolute blood counts of full Wt and Neo1 gt//gt chimeras after 15 months; n = 7 (Ctrl)–11 (Neo1), two independent experiments, for HB: 4 (Ctrl)–7 (Neo1). d Frequencies of B cells and myeloid cells of C45.2 + cells in peripheral blood of Wt and Neo1 gt//gt chimeras after 15 months; n = 5–13 (for exact n /timepoint please see Source data file), two independent experiments. Analysis with two-way-ANOVA, multiple comparisons with LSD Fisher’s test. e Workflow: assessment of HSC potency derived from 15 months (aged) chimeras. f Frequency of CD45.2 + vs. competitor HSCs 16 weeks transplantation of 100 or 500 HSCs from of aged Wt and Neo1 gt//gt chimeras; n = 6 (Ctrl + 500 HSC Neo1)–7(100 HSC, Neo1), two independent experiments. g Workflow: secondary and tertiary transplantations of 15 months (aged) chimeras. h Absolute frequencies of bone marrow CD45.2 + HSPCs in 2° transplantations of aged Wt and Neo1 gt//gt chimeras after 4 months; n = 7 (Ctrl)–8 (Neo1), two independent experiments. i Absolute frequencies of bone marrow CD45.2 + HSPCs in 3° transplantations of aged Wt and Neo1 gt//gt chimeras after 4 months; n = 6, two independent experiments. j Workflow: generation of full chimeras used in ( k – m ). k Cell cycle phase of CD45.2 + HSCs derived from Wt and Neo1 gt//gt chimeras after 4 months; n = 4 (Ctrl)–6 (Neo1), two independent experiments. l MFI of CDK6 in CD45.2 + HSC derived from Wt and Neo1 gt//gt chimeras after 4 months; n = 23 (Neo1)–29 (Ctrl). m Frequency of BrdU + CD45.2 + HSC derived from Wt and Neo1 gt//gt chimeras after 4 months, 48 h post BrdU injection; n = 6, two independent experiments. For all panels, ±SD is shown. n indicates biological replicates. P value was determined by two-tailed t test unless stated otherwise. Scale bars in IF images are 5 μm. Source data are provided as a Source Data file. Full size image Molecular signatures of activation and HSC dysfunction are enriched in Neo1- mutant HSCs To understand the molecular basis for the disruption of long-term self-renewal caused by loss of Neo1, we performed RNA-sequencing (RNA-seq) analysis of Neo1 gt/gt and wild-type (Wt) CD45.2 + HSCs 4 months (expanding Neo1 -mutant HSCs) and 15 months (exhausted Neo1 -mutant HSCs) after transplantation (Fig. 4a and Figure S 2a ). The principal component analysis showed the main mode of transcriptional variation to be attributable to age. The molecular consequences of mutant Neo1 were recapitulated by PC-2 and the difference increased upon ageing (Fig. 4a and Figure S 2b ). As expected, Neo1 expression itself was diminished in Neo1 -mutant HSCs, but interestingly strongly upregulated in aged compared to young Wt HSCs (Figure S2c ). Analysis of shared functional differences between young and old Neo1 -mutant HSCs compared to controls using Gene Set Enrichment Analysis (GSEA), we revealed cell cycle-associated gene sets like Hallmark(HM)_Mitotic_Spindle and HM_G2M_Checkpoint to be enriched in Neo1 mutants (Fig. 4b ) validating the functional data. This pattern of increased activation in Neo1 -mutant HSCs was also observed employing HSC-specific cell cycle signatures [49] (Fig. 4b ). In line with these data, the signature for aHSCs was enriched in Neo1 -mutant HSCs, in turn the signature for dHSCs was enriched in Wt HSCs [11] (Fig. 4b ). Reflecting the observed functional deficits of Neo1 -mutant HSCs, the MoIO [50] signature associated with superior HSC function was overrepresented in Wt HSCs, while the NoMO signature [50] , enriching for less quiescent, functionally inferior HSCs were enriched in Neo1 -mutant HSCs (Fig. 4b ). Analysis of differentially expressed genes (DEGs) identified genes associated with differentiation such as Itga2b and Gata1 [50] , [51] , [52] , as well as cell cycle regulators such as Cdk6 [53] (Fig. 4c and Figure S 2f ) or Mki67 (Figure S2d ) to be upregulated in Neo1 -mutant HSCs. In contrast, genes known to regulate HSC self-renewal or quiescence, such as Egr1 [54] , [55] , Zfp36 [56] and c- Fos [57] were downregulated (Fig. 4c and Figure S 2f ). Interestingly, Cdk6 has been shown to suppress Egr1 expression during HSC activation, which was suggested to promote HSC quiescence based on genetic data and thus is a likely downstream target of Neo1 [54] . No other Ntn1 receptors were differentially expressed (Figure S2e ). Therefore, the molecular data support the functional findings by revealing footprints of both loss of quiescence and diminished expression of HSC self-renewal related genes in Neo1 -mutant HSCs. In addition, we found that HSC ageing signatures [20] were enriched in Neo1 -mutant HSCs reflecting the observed functional decline (Fig. 4d ). In line, Klf6 , which has been proposed to maintain features of young HSCs in human, was downregulated in Neo1 -mutant HSCs [58] (Fig. 4e and Figure S 2f ). Finally, we report gene sets associated with nuclear factor-κB (NF-κB) signalling, as well as signalling of the NEO1 ligand netrin-1 (Ntn1) to be depleted in Neo1 -mutant HSCs, suggesting that these signalling pathways may be downstream of NEO1 activation (Fig. 4f ). Fig. 4: Neo1-mutant HSCs reveal a loss of quiescence and potency signatures. a , Left: workflow for RNA-seq of CD45.2 + HSCs from Wt and Neo1 gt//gt chimeras after 4 and 15 months. Right: sparse PCA; n = 2 (WT old/young, Neo1 young)–3 (Neo1 old). b GSEA for cell cycle and HSC potency of Wt vs. Neo1 gt//gt HSCs. FDR < 0.05, NOM p value <0.05. c Normalized read counts of DEG in HSCs from young and old Wt and Neo1 gt//gt chimeras, n = 4 (Ctrl)–5 (Neo1). d GSEA for HSC ageing signatures in Wt vs. Neo1 gt//gt HSCs. FDR < 0.05, NOM p value <0.05. e Normalized read counts of Klf6 in HSCs from young and old Wt and Neo1 gt//gt chimeras, n = 4 (Ctrl)–5 (Neo1). f GSEA for signalling pathways in Wt vs. Neo1 gt//gt HSCs. FDR < 0.05, NOM p value <0.05 . For all panels, ±SD is shown. n indicates biological replicates. Scale bars in IF images are 4 μm. P value was determined by two-tailed t test unless stated otherwise. Source data are provided as a Source Data file. Full size image Interestingly, when we tested enrichment for the Reactome_Netrin-1_Signalling gene set on RNA-seq data of a recent study of HSPC [1] , it was enriched in HSCs compared to all MPP populations, suggesting that Ntn1 signalling is physiologically active in homeostatic HSCs (Figure S2g ). In summary, we discover molecular features of both loss of quiescence and loss of self-renewal in Neo 1-mutant HSCs, paralleling functional results. NTN1 maintains HSC engraftment potential and quiescence via NEO1 signalling Next, we assessed whether the NEO1 ligands NTN1, RGM-a and RGM-b alone or in combination with their co-ligand BMP-2 were able to affect HSC behaviour. Because neither RGM s and Ntn1 nor additional Ntn1 receptors were expressed in HSCs (Figure S2h ) [1] , we sorted and cultured HSCs in the presence of NTN1, RGM-A and RGM-B with or without BMP-2 (Fig. 5a ). To assess active NEO1 signalling, we monitored Egr1 expression, which was downregulated in Neo1 -mutant HSCs (Fig. 5b ). After 48 h of stimulation, only NTN1, but none of the other ligands, induced expression of Egr1 (Fig. 5b ). This induction was absent in Neo1 -mutant HSCs (Fig. 5b ). 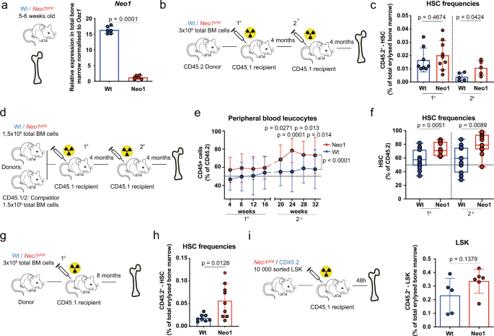Fig. 2: Mutant Neo1 causes an initial HSC expansion. aRelative expression ofNeo1in the total bone marrow of Wt andNeo1gt/gtmice;n= 6, three independent experiments.bWorkflow: generation of full chimeras.cAbsolute frequencies of bone marrow CD45.2+HSCs in full Wt andNeo1gt/gtchimeras 4 months after first and second transplantation;n= 5 (2nd Tx)–8 (Ctrl 1st Tx) and 9 (Neo1 1st TX), two independent experiments.dWorkflow: competitive transplantations.ePeripheral blood CD45.2+chimerism during 1° and 2° competitive transplantations of Wt andNeo1gt/gtbone marrow;n= 13–17 (for exactn/timepoint please see Source data file), three independent experiments, Analysis with two-way ANOVA, multiple comparison with LSD Fisher’s test.fCD45.2+chimerism of HSCs at endpoints of 1° and 2° competitive transplantations of Wt andNeo1gt//gtbone marrow;n= 11 (2nd TX), 12 (Ctrl 1st Tx), 14(Neo1 1st TX), three independent experiments. Whiskers are min–max, box is 25–75th percentile and line is mean.gWorkflow: full chimeras studied in (h).hAbsolute frequencies of bone marrow CD45.2+HSCs in full Wt andNeo1gt//gtchimeras after 8 months;n= 8 (Ctrl)–9 (Neo1), three independent experiments.iWorkflow: Homing assay in (j).jAbsolute frequencies of CD45.2+bone marrow LSK cells 48 h after transplantation of 10,000 sorted Wt andNeo1gt//gtLSK;n= 5 (Ctrl)–6 (Neo1). For all panels, ±SD is shown.nindicates biological replicates.Pvalue was determined by two-tailedttest unless stated otherwise. Source data are provided as a Source Data file. In addition, we detected a Neo1-dependent decrease in G2–S–M and an increase in G0-phase HSCs as well as diminished CDK6 protein levels (Fig. 5c, d ), paralleling the data from Neo1 -mutant HSCs in vivo (Fig. 4c, g ). We further confirmed the induction of quiescence by NTN1 with HSCs isolated from FUCCI [59] and c-Myc - GFP mice [60] reporter mice (Figure S2i, j ). Gene sets associated with NF-κB signalling were downregulated in Neo1 -mutant HSCs. Since NF-κB is essential for HSC maintenance and known to protect HSCs from premature differentiation upon stress [61] , we hypothesized that NTN1 may induce NF-κB signalling. To test this hypothesis, we isolated HSCs from p65-GFP mice, cultured them +/− NTN1 or +/− the p65 nuclear translocation inhibitor JSH-23 (Fig. 5e ). We observed increased nuclear p65 levels upon NTN1 treatment, which was blocked by JSH-23 (Fig. 5e ), suggesting that NTN1 maintains the canonical NF-κB pathway. We next assessed whether in vitro NTN1 stimulation translates into improved HSC engraftment in vivo. For this purpose, we stimulated 500 HSCs derived from either CD45.2 or CD45.1/2 mice with or without Ntn1 for 48 h, mixed treated with untreated congenically distinct HSCs and transplanted them into lethally irradiated recipients (Fig. 5f ). Four months after transplantation, we found increased engraftment of HSCs cultured with NTN1 in the BM, independent of genotype (Fig. 5g ). This showed that ex vivo treatment with NTN1 robustly improved the in vivo function of cultured HSCs. This effect of NTN1 was dependent on the presence of NEO1 since it was absent in Neo1 -mutant HSCs (Figure S2k ). Collectively, these data suggest that the NTN1–NEO1 axis preserves NF-κB activity, quiescence and in vivo function of cultured HSCs. Fig. 5: Ntn1 preserves HSC quiescence and engraftment potential in vitro via Neo1. a Workflow: In vitro stimulation of sorted HSCs used in ( b – d ), analysis after 48 h. b Relative expression of Egr1 in Wt HSCs; n = 3 (other), 4 (RGM-a + b), 16 (Ctrl/Neo1), for ctrl/Ntn1, four independent experiments. c Representative cell cycle plots pre-gated on HSCs and quantification with or without Ntn1 treatment; n = 3 (Neo1), 11 (Wt-Ctrl), 12 (Wt-Ntn1), three independent experiments for ctrl HSC. d MFI of CDK6 in Wt HSCs 48 h after Ntn1 treatment, quantification of MFI per cell; n = 114 (Ctrl) and 134 (Ntn1). e Workflow: representative images and quantification of total cell/nuclear MFI of p65-GFP HSC 48 h after treatment with Ntn1 or Ntn1 + JSH-23; n = 8 (JSH-23), 78 (Ctrl), 91 (Ntn1), two independent experiments. f Workflow: competitive transplantation of Ntn1 stimulated CD45.2 and CD45.1/2 HSCs. g Chimerism of bone marrow LSK-SLAM cells 4 months after competitive transplantation of Control vs. Ntn1-treated HSCs; n = 6 (CD45.1/2), 7 (CD45.2), two independent experiments. For all panels, ±SD is shown. n indicates biological replicates. Scale bars in IF images are 4 μm. P value was determined by two-tailed t test unless stated otherwise. Source data are provided as a Source Data file. Full size image Conditional Ntn1 deletion depletes HSCs and leads to activation and differentiation in vivo Next, we addressed the role of Ntn1 in hematopoiesis in vivo. Mice homozygous for an Ntn1-null allele ( Ntn1 β-geo/ β -geo ) die perinatally due to defects in cerebral development [62] and heterozygous mice display no hematopoietic phenotype (Figure S3a ). Therefore, we generated CAGGS:Cre ERT2 ; Ntn1 flox/flox mice [63] , [64] , which allows tamoxifen (Tam)-inducible ubiquitous deletion of Ntn1 (Figure S3h ). We induced deletion of Ntn1 at 6 weeks after birth ( Ntn1 ΔCAGGSCre/ΔCAGGSCre ) and analysed mice 8 weeks later (Fig. 6a ). Ntn1 deletion caused an increase in the relative frequencies of myeloid cells, especially neutrophils in both peripheral blood and BM (Figure S3b–d ). Strikingly, the frequency of HSCs in Ntn1 ΔCAGGSCre/ΔCAGGSCre BM was significantly reduced, while simultaneously the frequency of both MPP2 and MPP3/4 cells expanded (Fig. 6b, c and Figure S 3e, f ). In response to the induced Ntn1 deletion, HSCs entered a more proliferative, less quiescent state, represented by an increase of HSCs in G2–S–M and a reduction in G0 (Fig. 6d ). After Ntn1 deletion, HSCs also expressed reduced levels of Egr1 , while expression of Cdk6 , as well as the differentiation associated genes Gata1 and Itga2b increased (Fig. 6e ). Finally, Neo1 expression was upregulated in Ntn1 ΔCAGGSCre/ΔCAGGSCre HSCs, suggesting a compensatory upregulation in response to the absence of its ligand (Fig. 6e ). Fig. 6: In vivo Ntn 1 deletion depletes HSC and Ntn1 overexpression increases HSC quiescence. a Workflow: analysis of Ntn1 flox/flox and CAGGS:Cre ERT2 ; Ntn1 flox/flox mice 8 weeks after Cre induction for ( b – e ). b Representative flow cytometry plots of the LSK population of Ntn1 flox/flox and Ntn1 ΔCAGGS/ΔCAGGS mice. c Frequencies of bone marrow HSCs in Ntn1 flox/flox and Ntn1 ΔCAGGS/ΔCAGGS mice; n = 7 (flox)–10 (∆CAGGS), two independent experiments. d Cell cycle phase of HSCs derived from Ntn1 flox/flox and Ntn1 ΔCAGGS/ΔCAGGS mice; n = 8 (flox) and 10 (∆CAGGS), two independent experiments. e Relative expression of quiescence and activation related genes in HSCs derived from Ntn1 flox/flox and Ntn1 ΔCAGGS/ΔCAGGS mice; n = 6 (flox)–9 (∆CAGGS), two independent experiments. f Frequencies of bone marrow HSCs in Ntn1 flox/flox and Ntn1 ΔCAGGS/ΔCAGGS mice 5 months after Cre induction; n = 8 (∆CAGGS) and 12 (flox), three independent experiments. g Cell cycle phase of HSCs derived from Ntn1 +/LSL-Rosa26-Ntn1 and Ntn1-OE mice; n = 8 (∆CAGGS) and 12 (flox), three independent experiments. h Workflow: competitive transplantation of CAGGS:Cre ERT2 , Ntn1 ΔCAGGS/ΔCAGGS and Ntn1-OE mice 5 months after Cre induction, analysed in ( i – k ). i Representative FACS plots of peripheral blood leucocytes pre-gated on CD45 + cells at 16 weeks after transplantation. j Peripheral blood CD45.2 + chimerism during competitive transplantations; n = 13 (OE)–14 (Cre/∆CAGGS), two independent experiments. Analysis was done with two-way-ANOVA, multiple comparison with LSD Fisher’s test. k Bone marrow HSC CD45.2 + chimerism after 16 weeks of competitive transplantation; n = 12 (Cre)–13 (∆CAGGS/OE), two independent experiments. l Workflow: transplantation of 200 HSCs sorted from CAGGS:Cre ERT2 and Ntn1 ΔCAGGS/ΔCAGGS mice at 5 months after Cre induction. m Frequencies of bone marrow HSCs 8 weeks transplantation; n = 6. For all panels, ±SD is shown. n indicates biological replicates. P value was determined by two-tailed t test unless stated otherwise. Source data are provided as a Source Data file. Full size image The observed reduced numbers of HSCs were even more pronounced at 5 months post Ntn1 deletion, suggesting a progressive loss of HSCs after Ntn1 deletion (Fig. 6f and Figure S 3g, i ). To test whether increased levels of NTN1 could alter HSC behaviour in vivo, we generated CAGGS:Cre ERT2 ; LSL-Rosa26-Ntn1 mice ( Ntn1-OE ) and induced Cre expression in 6-week-old animals, leading to a 30-fold increase of Ntn1 levels in BM endothelial cells after 5 months (Figure S3h ). While we found no difference in HSPC frequencies (Figure S3j ), quiescent G0-HSCs increased, suggesting that Ntn1 overexpression in the BM microenvironment leads to increased HSC quiescence in vivo (Fig. 6g and Figure S 3k ). In addition, the frequency of cycling HSCs 5 months after Ntn1 deletion was significantly increased, reproducing the 2-month timepoint (Fig. 6d, g and Figure S 3k ). In summary, Ntn1 mediates HSC quiescence not only in culture but also in vivo and loss of Ntn1 activates and progressively depletes quiescent, functional HSCs. Conditional Ntn1 deletion impairs HSC function To study, whether the Ntn1-mediated increase ( Ntn1-OE ) or reduction in HSC quiescence and frequency ( Ntn1 deletion) is associated with functional consequences, we competitively transplanted total BM of Ntn1-OE, Ntn1 ΔCAGGSCre/ΔCAGGSCre or control ( CAGGS-Cre ERT2 ) mice 5 months after Tam induction (Fig. 6h ). Upon Ntn1-OE , we neither observed any differences in peripheral blood leucocytes nor in HSC frequencies 4 months after transplantation (Fig. 6i, k ). In contrast, Ntn1 deletion led to a reduced contribution of CD45.2 + donor cells to peripheral blood leucocytes (Fig. 6i, j ) accompanied with a strong reduction of HSC numbers 4 months after transplantation (Fig. 6k ). Next, we addressed the engraftment potential of 200 purified HSCs (LSK, CD150 + , CD48 − , CD34 − ) isolated either from a microenvironment, in which Ntn1 was deleted for 5 months ( Ntn1 ΔCAGGSCre/ΔCAGGSCre ) or expressed on normal levels (Fig. 6l ). Two months post transplantation, the HSC frequency was significantly reduced compared to control HSC, which have developed in an Ntn1-proficient environment (Fig. 6m ). These data show that HSCs derived from an Ntn1 -deficient BM become functionally impaired and this self-renewal defect is not reversed by transplanting them back into an Ntn1-proficient recipient microenvironment. Ntn1 expressed by arterioles maintains HSCs We next investigated which niche cells express Ntn1 . By screening published datasets, we found that Ntn1 is expressed at low levels in sinusoidal (SEC: CD45 − , CD31 + , Sca-1 medium , Pdpn + ) and at higher levels in arteriolar endothelial cells (AEC: CD45 − , CD31 + , Sca-1 high , Pdpn − ) [65] . In addition, Ntn1 expression has been reported in periarteriolar smooth muscle cells (SMCs) [66] . To examine Ntn1 expression within the BM niche, we isolated AECs, SECs, CD45 + hematopoietic and RFP + cells derived from Sma-RFP ( smooth muscle actin-RFP ) reporter mice marking SMCs [67] (Figure S4a, b ). While we found no expression in CD45 + hematopoietic cells, we detected the highest Ntn1 levels in AECs and SMCs (Fig. 7a ). To investigate whether periarteriolar smooth muscle-derived Ntn1 regulates HSCs, we generated Sma-Cre ERT2 ; Ntn1 flox/flox mice, injected adult mice with Tam and studied HSCs 8 weeks after Cre induction. In line with depletion of HSCs upon global Ntn1 deletion, we detected a decrease in HSCs in Ntn1 ΔSmaCre/ΔSmaCre animals compared to controls (Fig. 7b ). This reduction was, however, not as strong as we observed upon global Ntn1 deletion using CAGGS-Cre (Fig. 6 ), suggesting additional Ntn1 sources like AECs. As BM arterioles deteriorate upon ageing, leading to the loss of HSC maintaining SCF [23] , [24] , we isolated SECs and AECs from young and old Wt mice and found diminished Ntn1 expression specifically in old AECs (Fig. 7c ). When we investigated Neo1 in aged HSCs, we found expression was still restricted to HSCs, but levels were significantly increased (Figure S4c ), in line with our RNA-seq data from aged Wt chimeras (Figure S2d ). To further confirm this, we performed RNA-seq of young and old LSK-SLAM cells. We found membrane-associated processes and receptors to be upregulated upon ageing (Figure S4d ). Specifically, Neo1 expression increased robustly on RNA and protein level in old HSCs (Fig. 7d, e ). Several studies have previously compared transcriptional profiles of young vs. old HSCs (using different marker combinations). However, the studies showed a wide variety of DEGs with little consistency (Figure S4e ). To identify consistently changed DEGs upon HSC ageing, we added 12 previously published transcriptome datasets of aged HSCs to our own study and performed a meta-analysis (Figure S4e ). In these 13 datasets, not a single DEG was shared among ten or more studies, again highlighting the heterogeneity. Nevertheless, 13 genes were consistently differentially expressed in eight to nine datasets (Fig. 7f ). Seven of these were receptors and one of these was Neo1 , suggesting that Neo1 is one of the most consistently upregulated genes found upon HSC ageing. Fig. 7: Loss of niche-derived Ntn1 induces Neo1 in HSC upon ageing. a Relative expression of Ntn1 in CD45 + cells, SEC, AEC and RFP + SMC derived from Sma-RFP mice; n = 4 (CD45/AEC), 6 (SEC) and 7 (SMA-RFP), two independent experiments. b Frequencies of HSCs in bone marrow of in Ntn1 flox/flox and Ntn1 ΔSma/ΔSma mice; n = 8 (flox) and 10 (∆SMA), three independent experiments. c Relative expression of Ntn1 in SEC, AEC and CD45 + cells derived from young and old Wt mice; n = 3 (yCD45/oAEC), 4 (oSEC), 6 (ySEC) and 7 (yAEC), three independent experiments. d Normalized read counts of Neo1 in young, and old LSK-SLAM cells; n = 5 (young) and 7 (old), FDR < 0.0001. e MFI of NEO1 in sorted 6 or 24 months LSK-SLAM cells; n = 592 (young)–593 (old). f Most abundant common DEGs in published ageing studies and own data, additional details in the “Methods” section. g Relative expression of Neo1 in LSK-SLAM cells isolated from either denervated or healthy legs of individual mice; n = 8, two independent experiments. h Relative expression of Neo1 in HSCs of aged mice, before and after 2 months post transplantation; n = 6 (before) and 8 (after), two independent experiments. i Model of Neo1/Ntn1 axis in young and old mice. For all panels, ±SD is shown. n indicates biological replicates. Scale bars in IF images are 5 μm. P value determined by two-tailed t test unless stated otherwise. Source data are provided as a Source Data file. Full size image It has recently been established that surgical BM denervation mirrors the phenotype of arteriolar degeneration upon ageing and thereby induces premature HSC ageing [24] . Therefore, we tested whether the observed Neo1 upregulation during HSC ageing (Fig. 7d ) or as a consequence of Ntn1 deficiency (Fig. 6e ) was recapitulated upon denervation-mediated induction of premature marrow ageing. One hind limb per Wt mouse was surgically denervated and LSK-SLAM cells 4 months after surgery were analysed. We found an increase in Neo1 expression in HSCs of seven out of eight denervated femurs compared to sham-operated nerve-intact contralateral femurs of the same mice (Fig. 7g ). The Neo1 upregulation is consistent with a model that the normal or accelerated ageing process leads to a decrease in Ntn1 expression in the microenvironment, mediating a compensatory Neo1 upregulation to maintain signalling when its ligand Ntn1 becomes limiting. Finally, we investigated whether the niche mediated upregulation of Neo1 in HSCs of 30-month-old mice (NTN1 low environment) can be reversed by transplanting them into 2-month-old young mice (NTN1 high environment). Indeed, Neo1 expression in HSCs significantly decreased again in young mice (Fig. 7h ). These data further support the link between the level NTN1 production in the BM microenvironment and expression of its receptor Neo1 on HSCs in young and old mice (Fig. 7i ). However, the compensatory upregulation of Neo1 expression due to age-dependent ligand deprivation is not sufficient to maintain NEO1 function, since ablation of either Ntn1 or Neo1 leads to proliferation and decreased self-renewal of HSCs, a hallmark of aged HSCs. Here, we identify arteriolar niche-derived NTN1 ligand and its cognate HSC-specific receptor NEO1 as a novel ligand-receptor signalling axis regulating HSC quiescence and long-term self-renewal. This axis is deregulated upon ageing and loss of either of its components leads to functional HSC impairment. NTN1–NEO1 represents a novel intercellular and non-cell autonomous signalling network by which NTN1 produced by perivascular niches binds to HSCs to fine-tune HSC dynamics, in particular cell cycle activity and long-term self-renewal. In agreement with Neo1 being specifically expressed by dHSCs (Fig. 1 ), Neo1 is part of the MoIO signature marking functionally superior HSCs [50] . Expression of Neo1 is also highest in Vwf + HSCs residing on the top of the hematopoietic hierarchy [68] and NEO1 + cells have recently been reported as a subpopulation within Hoxb5 + HSCs [42] . Intriguingly, Dnmt3a mutant HSCs show increased quiescence, as well as a robust upregulation of Neo1 expression [69] , [70] , [71] , suggesting it as a potential target for Dnmt3a mutant hematopoietic disorders. When characterizing Neo1 -mutant hematopoiesis, we observed an initial increase in HSC numbers associated with loss of quiescence and subsequently loss of HSC self-renewal over time that correlated with decreased expression of Egr1 and increased expression of Cdk6 . Similarly, hematopoietic loss of Egr1 leads to increased cycling and initial HSC expansion followed by a loss of engraftment potential upon serial transplantation [55] . Since we analysed a hypomorphic Neo1 mouse model with severely decreased (>90%) but remaining minor expression [38] , [47] , [48] , our results possibly underestimate the biological relevance of Neo1 in HSCs. It has been reported, that ≈80% of Neo1 gt/gt mice die prenatally. The ones born develop hydrocephalus of varying degree, with around one in five displaying severe phenotypes with macroscopically visible “dome-shaped” skulls [48] . Since this was reproducible in our analysis, we used only Neo1 gt/gt mice without macroscopic features of hydrocephalus, which showed normal, healthy behaviour. In these Neo1 gt/gt mice, the HSC numbers were unchanged at the time of analysis. Nevertheless, we cannot formally exclude that additional factors such as neuronal stress may contribute to some extent to the described HSC phenotype in the primary Neo1 gt/gt mutants. NEO1 can bind multiple neural guidance molecules, which mediate context-dependent effects. As an example, RGMs are known to inhibit neuronal migration [72] , while NTN1 acts as a chemoattractant for commissural axons [63] . In HSCs, we found NTN1, but neither RGMs nor BMP-2, to modulate HSC behaviour. This is intriguing because, in the developing bone, NEO1 modulates cartilage growth via canonical BMP signalling [73] . However, the relevance of BMP signalling for adult HSCs remains uncertain [74] . Over the past years, the role of netrins in neurobiology, originally established using gene-trapped mice [62] , has been challenged by novel conditional Ntn1 alleles [63] , [75] , [76] . When we repurposed these to investigate hematopoiesis, we found increased activation and progressive loss of HSC numbers as well as self-renewal potential after global deletion of Ntn1 , mimicking the Neo1 -mutant phenotype. Further, in vivo overexpression and in vitro stimulation with NTN1 enhanced HSC quiescence and increased engraftment potential of cultured HSCs upon transplantation, respectively. These results are in line with studies showing quiescence-inducing compounds that maintain HSC engraftment potential in vitro [11] , [29] , [77] as well as studies that associate loss of self-renewal capability in vivo with divisional history [13] , [78] , [79] . Altogether, the data strongly suggest that NTN1 acts as a paracrine NEO1 ligand modulating HSC behaviour. Furthermore, Ntn1 has been described to support immature states of iPSCs and cancer stem cells [80] , [81] , suggesting that it maintains stemness in various settings. Here, we demonstrate that NTN1/NEO1 signalling increase NF-κB activation in HSCs, a pathway known to protect HSCs from exhaustion during stress, while the loss of p65 leads to hematopoietic failure [61] , [82] . Within the BM niche, we found Ntn1 to be expressed in AECs and SMC in line with the previous studies [65] , [83] , [84] . These as well as other perivascular cells secrete multiple molecules that support HSCs including SCF and CXCL12 [26] , [27] , [65] , [83] , [85] , [86] . Upon ageing, BM arterioles are remodelled leading to a depletion of periarteriolar stromal cells and SCF, affecting hematopoiesis [23] , [24] , [25] . In line, NTN1 secretion by SMCs is known to guide axons of the sympathetic nervous system during arteriolar growth [66] . The connection between the sympathetic nervous system and arterioles is intriguing, as denervation disrupts BM arterioles and mediates accelerated HSC ageing [24] . Our data strongly support the link between NTN1 production in the BM microenvironment and expression of its receptor Neo1 on HSCs. Loss of Ntn1 expression in the niches during: (a) physiological ageing, (b) accelerated ageing by surgical denervation or (c) by genetic ablation results in compensatory upregulation of Neo1 expression due to ligand deprivation, which, however, is not sufficient to maintain Neo1 function. Such a mechanism has also been observed for the Ntn1 receptors DCC and NEO1 upon loss of Ntn1 during development [76] . Collectively, our data suggest that NTN1 produced mainly by arteriolar niches preserves quiescence and self-renewal of HSCs via NEO1, while ageing-associated decline of Ntn1 leads to the gradual decrease of Neo1-mediated HSC self-renewal. Contact for reagent and resource sharing Further information and requests for resources and reagents should be directed to and will be fulfilled by the Lead Contact, Andreas Trumpp a.trumpp@dkfz.de. Certain materials are shared with research organizations for research and educational purposes only under an MTA to be discussed in good faith with the recipient. Experimental mouse models SCL-tTA; H2B-GFP mice This transgenic mouse line expresses the fusion protein histone H2B-GFP under the tetracycline-responsive regulatory element and the tTA-S2 transactivator from the endogenous Scl locus [10] . Doxycycline was supplemented in drinking water of 8–16-week-old mice for 150 as previously described [10] . To set the gates for GFP + cells, age-matched H2B-GFP littermates were used. SCL-tTA; H2B-GFP mice were backcrossed to C57BL/6J. C57BL/6J (CD45.2, CD45.1 or CD45.2/CD45.1) mice were either purchased from Envigo (the Netherlands) or Janvier Labs (France) or bred in-house. Gprc5c-GFP mice ( Tg(Gprc5c-EGFP)JU90Gsat ) This transgenic mouse line was previously generated by inserting an EGFP gene into a BAC clone at the initiating ATG codon of the first coding exon of the Gprc5c gene and this BAC clone was subsequently used to generate transgenic reporter mice [87] . Analysed mice were backcrossed to C57BL/6J. Myc-eGFP mice This transgenic mouse line expresses a fusion protein of c-Myc and eGFP [60] . FUCCI mice (B6-Tg(Gt(ROSA)26Sor-Fucci2)#Sia ) This transgenic mouse line allows the identification of cell cycle phase via fluorescent fusion proteins, mice were sacrificed after 8–16 weeks [59] . Neo1 gt/gt mice ( B6.129P2-Neo1 Gt(KST265)Byg/Mmmh ) These mice harbour a gene-trapped Neo1 allele that leads to a strong reduction of Neo1 expression [38] . For transplantation experiments, male and female animals 4–6 weeks of age were used. Control transplantations were always performed using gender-matched, wild-type littermates. For competitive transplantations, competitor BM was also age- and gender-matched. Ntn1 β-geo/+ mice ( Ntn1 Gt(ST629)Byg ) These mice harbour a gene-trapped Ntn1 allele that leads to a strong reduction of Ntn1 . Heterozygous mice can be used as reporter mice employing the β-gal reporter in the gene-trapped vector [62] . Ntn1 fl/fl mice This transgenic mouse line contains loxP sites flanking coding sequences containing both the principal ATG (based on Ntn1 complementary DNA (cDNA) sequence NM_008744) and the cryptic ATG (based on Ntn1 cDNA: BC141294) and the alternative promoter described in intron 3 [63] . To generate global Ntn1 deletion, we crossed Ntn1 fl/fl mice to CAGGS-Cre ERT2 mice (Jackson Laboratories). For smooth muscle-specific deletion, Ntn1 fl/fl mice were crossed to Sma-Cre ERT2 mice. For 8 weeks endpoints, Ntn fl/fl crossings only female, and for 5 months endpoints, only male mice were analysed to reduce variability. +/LSL-Rosa26-Ntn1 mice This transgenic mouse line was generated for this study. The human NETRIN-1 was cloned in Rosa26-lox-stop-lox plasmid (Soriano). Mice were generated by SEAT CNRS Gustave Roussy Phenomin. We crossed these mice to CAGGS:Cre ERT2 mice (Jackson Laboratories), inducing global overexpression of Ntn1. To reduce variability, only male animals were analysed at 5 months after Cre induction. Sma-RFP mice ( C.Cg-Tg(aSMA-RFP)#Rkl The mouse line harbours an RFP reporter for Sma and thereby allows identification of SMCs [67] . Sma-RFP mice are on a BALB/C background. All other mouse models are on a B6J background. All mice were bred in-house in the animal facilities of DKFZ, University Medical Center Groningen, INSERM or Albert-Einstein College of medicine under specific pathogen-free conditions in individually ventilated cages at 24°, a humidity of 80% with fixed day/night cycles of 12 h. According to German, French, American or Dutch guidelines, mice were euthanized by cervical dislocation and all animal procedures were performed according to protocols approved by the Regierungspräsidium Karlsruhe, Animal Care and Use Committee of Albert-Einstein College of Medicine, the Instantie voor Dierenwelzijn committee, Universitair Medisch Centrum Groningen/Rijksuniversiteit Groningen or University of Lyon local Animal Ethic Evaluation Committee. To reduce animal numbers, remaining BM/cDNA samples generated in this and previous studies were used whenever possible. Method details pIC- or LPS-induced inflammatory stress Mice were injected intraperitoneally with pIC (100 μg/mouse in 0.1 ml phosphate-buffered saline (PBS)), LPS (5 μg/mouse in 0.1 ml PBS) or PBS alone. Sixteen hours (LPS/pIC/PBS), 5 or 8 days (pIC/PBS) later, mice were sacrificed and BM cells were used for subsequent analysis. Cell isolation and flow cytometry Mouse BM cells were isolated, and HSCs and MPP1–4 progenitors defined by immune phenotype (lineage-negative (Lin − ), Sca-1 + , c-Kit + (LSK), CD135 −/+ , CD150 −/+ , CD48 −/+ , CD34 −/+ , CD45.2 CD45.1/2, CD45.1) (see also Fig. 1a ), or LSK-SLAM (Lin − c-Kit + CD150 + CD48 − ) purified by FACS and subsequently subjected to RNA-seq, population quantitative real-time PCR (qPCR) analysis, in vitro experiments, reconstitution assays or cytological analysis. Briefly, BM was isolated from pooled femora, tibiae, ilia and vertebrae by gentle crushing in PBS using a mortar and pistil. If no depletion of lineage-positive (Lin + ) cells was performed, lysis of erythrocytes was performed using ACK Lysing Buffer (Thermo Fisher Scientific). To deplete Lin + cells we used the Dynabeads Untouched Mouse CD4 Cells Kit (Invitrogen). Briefly, total BM was stained for 30 min with 100 μl/mouse of the Lineage Cocktail provided in the Dynabeads Untouched Mouse CD4 Cells Kit (Invitrogen) in PBS. Labelled cells were then incubated for 20 min with 1.5 ml/mouse of washed polyclonal sheep anti-rat IgG-coated Dynabeads provided in the Kit. Cells were depleted using a magnet, enriching for the Lin − cell fraction. To purify HSC and MPP1–4, the Lin − fraction was stained for 30 min using the following monoclonal antibodies: anti-lineage [anti-CD4 (clone GK1.5), anti-CD8a (53-6.7), anti-CD11b (M1/70), anti-B220 (RA3-6B2), anti-GR1 (RB6-8C5) and anti-TER119 (Ter-119)]; anti-CD117/c-Kit (2B8); anti-Ly6a/Sca-1 (D7); anti-CD34 (RAM34); anti-CD150 (TC15-12F12.2); anti-CD48 (HM48-1); anti-CD135 (A2F10); CD45.1 (A20); CD45.2 (104). The coupled fluorochromes used depended on the experiment to allow sorting of different fluorescent protein containing reporters or isolation of HSC from transplants. Monoclonal antibody conjugates were purchased from eBioscience, BD Bioscience or BioLegend. Cell sorting was then performed on a FACS Aria I, II and III, FACS Aria Fusion (Becton Dickinson) using BD FACSDiva v8.0.3 (BD Bioscience) or MoFlo Astrios or XDP cell sorters (Beckman Coulter). Sorted in Complete Stem Cell Medium (specified elsewhere) for in vitro culture, cytology and reconstitution experiments, or RNA lysis buffer (ARCTURUS PicoPure RNA Isolation Kit (Life Technologies, Invitrogen) for population RNA-seq or qPCR and stored at −80 °C. For Figure S4c , long-term HSCs were characterized as Lin − Sca-1 + c-Kit + CD48 − CD150 + , ST-HSCs as Lin − Sca-1 + c-Kit + CD48 − CD150 − and MPPs as Lin − Sca-1 + c-Kit + CD48 + CD150 − . For isolation of committed progenitor subsets, the following markers were used for isolation: CLP (Lin − CD127 + Sca-1 lo c-Kit lo ), CMP (Lin − CD127 − Sca-1 − c-Kit − CD34 + CD16/CD32 hi ), GMP (Lin − CD127 − Sca-1-c-Kit + CD16/CD32 hi ) and MEP (Lin − CD127 − Sca-1 − c-Kit + CD34 − CD16/CD32 + ). Data were analysed using FlowJo, versions 6-10.5.3. CDK6/NEO1 staining For analyses of NEO1 expression, BM cells were isolated from mice and stained for HSC/MPP markers and sorted as described. Cells were plated on poly- l -lysine-coated slides and then fixed with BD Cytofix/Cytoperm Buffer (Beckton Dickinson). Subsequently, Cdk6 (Abcam) or Neo1 (Abcam) staining was performed in 0.1% Triton (Sigma) and 5% bovine serum albumin (BSA). Secondary antibodies coupled to AF-488 were used. After washing, slides were embedded in anti-fade reagent with 4′,6-diamidino-2-phenylindole (DAPI) (Invitrogen) and imaging was performed employing a Zeiss LSM 700 or LSM 710 confocal microscope using ZEN blue v2.5 (Zeiss international). Experimental replicates were always performed side by side and imaged in one session without change of laser intensities or gain to avoid technical bias and allow the comparability. DAPI signal was not used for quantification or normalization. The analysis was performed with FIJI v.2.0. NEO1 staining (Fig. 7e ) A total of 4000–6000 long-term HSCs were seeded in spots of an immunofluorescent adhesion slide (VWR) and allowed to settle for 20 min. Cells were then fixed and permeabilized with Fixation and Permeabilization Solution (BD Biosciences) for 20 min on ice. Cells were then blocked with 4% BSA for 30 min at room temperature and then stained with 1:100 mouse Neo1 biotinylated antibody (R&D) at 4 °C. Cells were washed three times in 0.1% Triton X-100 PBS solution and stained with 1:500 secondary antibody streptavidin Alexa-647 for 1 h at 4 °C. After washing, coverslips were mounted in anti-fade reagent with DAPI (Invitrogen). p65-GFP staining After 48 h of the culture of 2000 HSCs/well, cells were plated on poly- l -lysine-coated slides and then fixed with BD Cytofix/Cytoperm Buffer (Beckton Dickinson). Subsequently, anti-GFP-488 (Abcam) staining was performed in 0.1% Triton (Sigma) 5% BSA for 1 h to increase the signal. After washing, coverslips were mounted in anti-fade reagent with DAPI (Invitrogen). Cell cycle analysis HSC/MPP surface staining (LSK, CD150, CD48, CD34) was performed on BM cells or in vitro treated HSPCs. Cells were fixed with BD Cytofix/Cytoperm Buffer (Beckton Dickinson). Subsequently, intracellular Ki-67 (BD Biosciences) staining was performed using PermWash solution (Beckton Dickinson). Prior to flow cytometry analysis, cells were stained with Hoechst 33342 (Invitrogen) or DAPI (Thermo Fisher). Population RNA-seq For Fig. 4e–j and Figure S2c–e , population RNA-seq data were generated as previously described [1] . Briefly, total RNA isolation was performed using ARCTURUS PicoPure RNA Isolation Kit (Life Technologies, Invitrogen) according to the manufacturer’s instructions. Total RNA was used for quality controls and for normalization of starting material. cDNA libraries were generated using 1 ng of total RNA for Neo1 -deficient/Wt HSCs using the SMARTer Ultra Low RNA Kit for Illumina Sequencing (Clontech) according to the manufacturer’s indications. Sequencing was performed using the HiSeq2000 device (Illumina). RNA-seq: young and old LSK-SLAM for Fig. 7d and Figure S4d RNA was isolated from 15,000 LSK-SLAM cells (Lin − Sca-1 + c-Kit + CD48 − CD150 + ) using the Nucleospin XS Kit (Macherey Nagel) and quantified on Bionalyzer using RNA Pico 6000 Kit (Agilent). Ribosomal depletion was performed using a modified version of RiboZero Kit (Illumina). In all, 300 pg ribosomal-depleted RNA was used as input into TotalScript RNA-Seq Kit (Epicentre). Libraries were pooled and sequenced to 30–50 million reads on HiSeq 2500. qPCR analysis For qPCR, total RNA of 2000–10,000 cells were isolated as described above or using Nucleospin RNA XS Kit (Machery-Nagel) and reverse-transcribed using SuperScript VILO cDNA Synthesis Kit (Invitrogen) according to the manufacturer’s guidelines. For qPCR analysis, Fast SYBR Green Master Mix (Thermo Scientific) or LightCycler SYBR Green I (Roche) was used on a ViiA 7 Real-Time PCR System (Applied Biosystems) or a LightCycler 480 Instrument (Roche). RNA expression was normalized to Oaz1 , Act2b , or Hprt housekeeping gene expression and presented as relative quantification (ratio = 2 − DDCT ). Primers were designed using the Universal ProbeLibrary Assay Design Center (Roche) or NCBI Primer-BLAST (NCBI) and ordered from Sigma. Primer sequences are available in the Supplementary Information file. Reconstitution experiments For the generation of full chimeras, 3 × 10 6 total BM cells from 4-week-old Wt CD45.2 or Neo1 gt/gt CD45.2 mice were injected per recipient mouse. For the generation of 50/50 chimeras, 1.5 × 10 6 total BM cells from 4-week-old Wt CD45.2 or Neo1 gt/gt CD45.2 mice were mixed with 1.5 × 10 6 total BM cells derived from CD45.1/2 mice so that a total of 3 × 10 6 BM cells was injected per recipient mouse. For transplantation after in vitro treatment, 500 sorted HSCs of CD45.1/2 or CD45.2 derived from 8- to 12-week-old animals were cultured for 48 h in respective conditions. Then, a well of the progeny of CD45.1/.2 was mixed to a well of the progeny of CD45.2 and then transplanted. A similar setup was used for the assessment of Neo1 dependency of in vitro Ntn1 treatment: 500 Neo1 -deficient CD45.2 + HSCs were sorted after 8 months from old Neo1 full chimeras and then incubated with or without Ntn1. These Neo1- deficient HSCs were mixed with 500 CD45.1/2 HSC incubated without Ntn1, derived from 8-week-old CD45.1/2 animals and then transplanted into individual recipients. For secondary transplantations, 3 × 10 6 total BM cells were isolated and transplanted. For potency assessment of 100/500 CD45.2 Wt or Neo1- mutant HSCs were sorted from straight chimeras 15 months after transplantation, mixed with 1 × 10 5 total BM cells from 8- to 12-week-old CD45.1/.2 mice and transplanted. For assessment of HSC homing, 10 × 10 3 LSK cells derived from CD45.2 Wt or Neo1 -deficient mice were sorted and transplanted. For the generation of 50/50 chimeras, 1.5 × 10 6 total BM cells from 6.5-month-old Ntn1-OE/ Ntn1 ΔCAGGSCre/ΔCAGGSCre or CAGGS-Cre mice, were mixed with 1.5 × 10 6 total BM cells derived from CD45.1/2 mice so that a total of 3 × 10 6 BM cells was injected per recipient mouse. For transplantations of sorted HSC, 200 HSCs from 6.5-month-old Ntn1 ΔCAGGSCre/ΔCAGGSCre or CAGGS-Cre were mixed with 1 × 10 6 total spleen cells from CD45.1/2 mice and injected into the recipient. For transplantation of a 30-month-old HSC, 3 × 10 6 total BM cells were isolated and injected into recipients. For all experiments, cells were transplanted into fully irradiated (2 × 5 Gy) B6J mice (CD45.1). Contribution of CD45.2 or CD45.1/.2 donor cells was monitored in peripheral blood approximately every 4 weeks post transplantation in all transplantations using either LSRII, LSR Fortessa. Outcome was addressed by absolute blood counts or flow cytometry using the following monoclonal antibodies: anti-CD45.1 (A20); anti-CD45.2 (104); anti-CD4 (clone GK1.5), anti-CD8a (53-6.7), anti-CD11b (M1/70), anti-B220 (RA3-6B2), anti-GR1 (RB6-8C5). The applied fluorochromes depended on the experiment. For endpoint analysis of chimera animals, BM stainings were performed as following: anti-lineage [anti-CD4 (clone GK1.5), anti-CD8a (53-6.7), anti-CD11b (M1/70), anti-B220 (RA3-6B2), anti-GR1 (RB6-8C5) and anti-TER119 (Ter-119)]; anti-CD117/c-Kit (2B8); anti-Ly6a/Sca-1 (D7; anti-CD34 (RAM34); anti-CD150 (TC15-12F12.2−; anti-CD48 (HM48-1); anti-CD45.1 (A20); anti-CD45.2 (104)). Monoclonal antibody conjugates were purchased from eBioscience, BD Bioscience or BioLegend. Tam induction schema For Sma : Cre ERT2 ; Ntn1 fl/fl , CAGGS:Cre ERT2 ; Ntn1 fl/fl Ntn1 fl/fl and CAGGS:Cre ERT2 ; LSL-Rosa26-Ntn1 mice 3 Tam (Sigma-Aldrich) injections in 1 week were performed 4–6-week-old animals. At 8 weeks or 5 months after Cre induction mice were sacrificed and analysed. BrdU analysis Full chimeras of Neo1 -mutant or Wt CD45.2 BM were injected intraperitoneally with 0.2 ml BrdU (1.8 mg/ml; Sigma) 4 months after transplantation and sacrificed 48 h after injection. Then, HSC surface staining was performed as described above, cells were processed and then staining with anti-BrdU (BD Bioscience) antibody (1:30) was performed. HSPCs plating and in vitro treatment In all, 5000 LSK-SLAM cells for RNA analysis, or 5000–10,000 HSCs for imaging or cell cycle analysis were sorted into and then cultured in Complete Stem Cell Medium (StemPro-34 SFM, Life Technologies containing 50 ng/ml SCF and 25 ng/ml TPO (all Preprotech), 100 U/ml penicillin/streptomycin, 2 mM l -glutamine, StemPro-34 supplement as recommended). Cells were cultured in 96-well ultralow attachment plates (Corning) and were treated with either recombinant 1 μl/ml Ntn1 (R&D), 1 μl/ml Rgm-a (R&D), 1 μl/ml Rgm-b (R&D), or 200 ng/ml Bmp-2 (R&D) in addition to the standard cytokines. The concentration of JSH-23 was 6 μM. At 48 h after plating, cells were used for downstream procedures such as RNA isolation, imaging or flow cytometry as described in its respective chapter. BM denervation by the transaction of femoral and sciatic nerves Denervation of the femoral and tibial BM was done as previously described [24] . The femoral nerve was localized after its exit from the vertebral column deep in the psoas muscle. This was accomplished with a midline abdominal incision; the intestines were gently moved aside to visualize the psoas muscle. An incision was made in the psoas to visualize the femoral nerve, and a 1 cm section of the nerve was excised. Deep to the psoas (through the incision), the sciatic nerve was visualized in close proximity to the iliac crest of the pelvis, and a 1 cm section of the nerve was excised. For sham operation, both femoral and sciatic nerves were exposed by surgery, but were left intact. BM digestion for stromal cell isolation For isolation of stromal cells, we thoroughly cleaned dissected bones, crushed and digested them for 1 h in RPMI with 2% fetal calf serum as well as 0.25% collagenase Type I (Gibco). 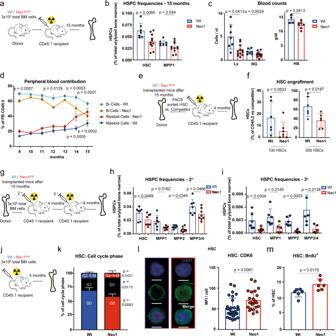Fig. 3: Mutant Neo1 causes premature HSC exhaustion. aWorkflow: aged chimeras, analysed in (b–d).bAbsolute frequencies of bone marrow CD45.2+HSPCs in full Wt andNeo1gt//gtchimeras after 15 months;n= 7 (Ctrl)–11 (Neo1), two independent experiments.cAbsolute blood counts of full Wt andNeo1gt//gtchimeras after 15 months;n= 7 (Ctrl)–11 (Neo1), two independent experiments, for HB: 4 (Ctrl)–7 (Neo1).dFrequencies of B cells and myeloid cells of C45.2+cells in peripheral blood of Wt andNeo1gt//gtchimeras after 15 months;n= 5–13 (for exactn/timepoint please see Source data file), two independent experiments. Analysis with two-way-ANOVA, multiple comparisons with LSD Fisher’s test.eWorkflow: assessment of HSC potency derived from 15 months (aged) chimeras.fFrequency of CD45.2+vs. competitor HSCs 16 weeks transplantation of 100 or 500 HSCs from of aged Wt andNeo1gt//gtchimeras;n= 6 (Ctrl + 500 HSC Neo1)–7(100 HSC, Neo1), two independent experiments.gWorkflow: secondary and tertiary transplantations of 15 months (aged) chimeras.hAbsolute frequencies of bone marrow CD45.2+HSPCs in 2° transplantations of aged Wt andNeo1gt//gtchimeras after 4 months;n= 7 (Ctrl)–8 (Neo1), two independent experiments.iAbsolute frequencies of bone marrow CD45.2+HSPCs in 3° transplantations of aged Wt andNeo1gt//gtchimeras after 4 months;n= 6, two independent experiments.jWorkflow: generation of full chimeras used in (k–m).kCell cycle phase of CD45.2+HSCs derived from Wt andNeo1gt//gtchimeras after 4 months;n= 4 (Ctrl)–6 (Neo1), two independent experiments.lMFI of CDK6 in CD45.2+HSC derived from Wt andNeo1gt//gtchimeras after 4 months;n= 23 (Neo1)–29 (Ctrl).mFrequency of BrdU+CD45.2+HSC derived from Wt andNeo1gt//gtchimeras after 4 months, 48 h post BrdU injection;n= 6, two independent experiments. For all panels, ±SD is shown.nindicates biological replicates.Pvalue was determined by two-tailedttest unless stated otherwise. Scale bars in IF images are 5 μm. Source data are provided as a Source Data file. After digestion was stopped with 10% fetal calf serum-containing medium, red cell lyses, lineage depletion, staining and cell sorting were performed as described above. Quantification, statistics and reproducibility Standard quantifications, display and experimental design Statistical analysis was performed with two-tailed paired Student’s t test or two-way analysis of variance using Fisher’s least significant difference for multiple comparisons as indicated in the respective figure legend. 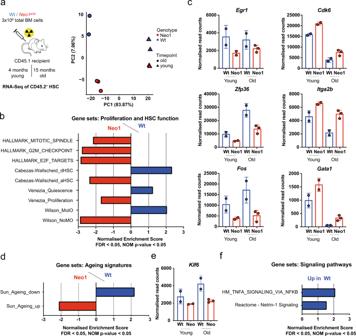Fig. 4: Neo1-mutant HSCs reveal a loss of quiescence and potency signatures. a, Left: workflow for RNA-seq of CD45.2+HSCs from Wt andNeo1gt//gtchimeras after 4 and 15 months. Right: sparse PCA;n= 2 (WT old/young, Neo1 young)–3 (Neo1 old).bGSEA for cell cycle and HSC potency of Wt vs.Neo1gt//gtHSCs. FDR < 0.05, NOMpvalue <0.05.cNormalized read counts of DEG in HSCs from young and old Wt andNeo1gt//gtchimeras,n= 4 (Ctrl)–5 (Neo1).dGSEA for HSC ageing signatures in Wt vs.Neo1gt//gtHSCs. FDR < 0.05, NOMpvalue <0.05.eNormalized read counts ofKlf6in HSCs from young and old Wt andNeo1gt//gtchimeras,n= 4 (Ctrl)–5 (Neo1).fGSEA for signalling pathways in Wt vs.Neo1gt//gtHSCs. FDR < 0.05, NOMpvalue <0.05.For all panels, ±SD is shown.nindicates biological replicates. Scale bars in IF images are 4 μm.Pvalue was determined by two-tailedttest unless stated otherwise. Source data are provided as a Source Data file. All data are presented as mean ± SD. For box and whiskers plots, error bars depict min to max values, the box is defined at 25–75th percentile and the median is marked with an additional line. Please see figure legends for detailed information. GraphPad Prism 7/8 was used for statistical analysis. The number of independent experiments is indicated in the respective figure legends. Sample exclusion was only done as a result of premature mouse death, infection or clear mistakes in sample processing. RNA-seq analysis For RNA-seq of Neo1-mutant and control HSCs, the following pipeline was used: sequenced read fragments were mapped to the mouse reference genome GRCm38 using STAR (STAR_2.6.1a) [88] . Expression counts estimates were generated using HTSeq (htseq-0.9.1) [89] . DESeq2 (DESeq2_1.20.0) [90] was used to test for differential expression; results were considered significant at a p .adj. value <0.05. The analysis was performed in R-studio v3.5.2 ( www.r-project.org ). 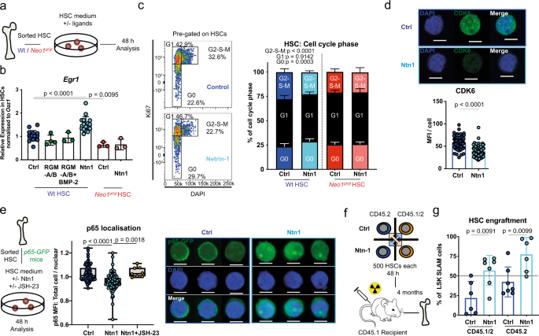Fig. 5: Ntn1 preserves HSC quiescence and engraftment potential in vitro via Neo1. aWorkflow: In vitro stimulation of sorted HSCs used in (b–d), analysis after 48 h.bRelative expression ofEgr1in Wt HSCs;n= 3 (other), 4 (RGM-a + b), 16 (Ctrl/Neo1), for ctrl/Ntn1, four independent experiments.cRepresentative cell cycle plots pre-gated on HSCs and quantification with or without Ntn1 treatment;n= 3 (Neo1), 11 (Wt-Ctrl), 12 (Wt-Ntn1), three independent experiments for ctrl HSC.dMFI of CDK6 in Wt HSCs 48 h after Ntn1 treatment, quantification of MFI per cell;n= 114 (Ctrl) and 134 (Ntn1).eWorkflow: representative images and quantification of total cell/nuclear MFI of p65-GFP HSC 48 h after treatment with Ntn1 or Ntn1 + JSH-23;n= 8 (JSH-23), 78 (Ctrl), 91 (Ntn1), two independent experiments.fWorkflow: competitive transplantation of Ntn1 stimulated CD45.2 and CD45.1/2 HSCs.gChimerism of bone marrow LSK-SLAM cells 4 months after competitive transplantation of Control vs. Ntn1-treated HSCs;n= 6 (CD45.1/2), 7 (CD45.2), two independent experiments. For all panels, ±SD is shown.nindicates biological replicates. Scale bars in IF images are 4 μm.Pvalue was determined by two-tailedttest unless stated otherwise. Source data are provided as a Source Data file. For Fig. 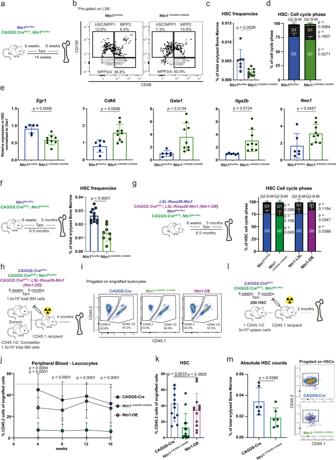Fig. 6: In vivoNtn1 deletion depletes HSC and Ntn1 overexpression increases HSC quiescence. aWorkflow: analysis ofNtn1flox/floxandCAGGS:CreERT2; Ntn1flox/floxmice 8 weeks after Cre induction for (b–e).bRepresentative flow cytometry plots of the LSK population ofNtn1flox/floxandNtn1ΔCAGGS/ΔCAGGSmice.cFrequencies of bone marrow HSCs inNtn1flox/floxandNtn1ΔCAGGS/ΔCAGGSmice;n= 7 (flox)–10 (∆CAGGS), two independent experiments.dCell cycle phase of HSCs derived fromNtn1flox/floxandNtn1ΔCAGGS/ΔCAGGSmice;n= 8 (flox) and 10 (∆CAGGS), two independent experiments.eRelative expression of quiescence and activation related genes in HSCs derived fromNtn1flox/floxandNtn1ΔCAGGS/ΔCAGGSmice;n= 6 (flox)–9 (∆CAGGS), two independent experiments.fFrequencies of bone marrow HSCs inNtn1flox/floxandNtn1ΔCAGGS/ΔCAGGSmice 5 months after Cre induction;n= 8 (∆CAGGS) and 12 (flox), three independent experiments.gCell cycle phase of HSCs derived fromNtn1+/LSL-Rosa26-Ntn1andNtn1-OEmice;n= 8 (∆CAGGS) and 12 (flox), three independent experiments.hWorkflow: competitive transplantation ofCAGGS:CreERT2,Ntn1ΔCAGGS/ΔCAGGSand Ntn1-OE mice 5 months after Cre induction, analysed in (i–k).iRepresentative FACS plots of peripheral blood leucocytes pre-gated on CD45+cells at 16 weeks after transplantation.jPeripheral blood CD45.2+chimerism during competitive transplantations;n= 13 (OE)–14 (Cre/∆CAGGS), two independent experiments. Analysis was done with two-way-ANOVA, multiple comparison with LSD Fisher’s test.kBone marrow HSC CD45.2+chimerism after 16 weeks of competitive transplantation;n= 12 (Cre)–13 (∆CAGGS/OE), two independent experiments.lWorkflow: transplantation of 200 HSCs sorted fromCAGGS:CreERT2andNtn1ΔCAGGS/ΔCAGGSmice at 5 months after Cre induction.mFrequencies of bone marrow HSCs 8 weeks transplantation;n= 6. For all panels, ±SD is shown.nindicates biological replicates.Pvalue was determined by two-tailedttest unless stated otherwise. Source data are provided as a Source Data file. 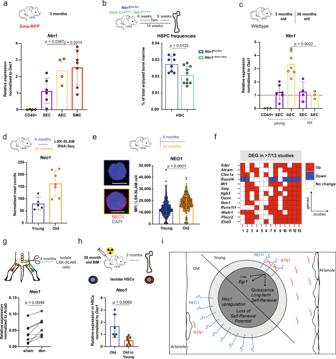Fig. 7: Loss of niche-derived Ntn1 induces Neo1 in HSC upon ageing. aRelative expression ofNtn1in CD45+cells, SEC, AEC and RFP+SMC derived fromSma-RFPmice;n= 4 (CD45/AEC), 6 (SEC) and 7 (SMA-RFP), two independent experiments.bFrequencies of HSCs in bone marrow of inNtn1flox/floxandNtn1ΔSma/ΔSmamice;n= 8 (flox) and 10 (∆SMA), three independent experiments.cRelative expression ofNtn1in SEC, AEC and CD45+cells derived from young and old Wt mice;n= 3 (yCD45/oAEC), 4 (oSEC), 6 (ySEC) and 7 (yAEC), three independent experiments.dNormalized read counts ofNeo1in young, and old LSK-SLAM cells;n= 5 (young) and 7 (old), FDR < 0.0001.eMFI of NEO1 in sorted 6 or 24 months LSK-SLAM cells;n= 592 (young)–593 (old).fMost abundant common DEGs in published ageing studies and own data, additional details in the “Methods” section.gRelative expression ofNeo1in LSK-SLAM cells isolated from either denervated or healthy legs of individual mice;n= 8, two independent experiments.hRelative expression ofNeo1in HSCs of aged mice, before and after 2 months post transplantation;n= 6 (before) and 8 (after), two independent experiments.iModel of Neo1/Ntn1 axis in young and old mice. For all panels, ±SD is shown.nindicates biological replicates. Scale bars in IF images are 5 μm.Pvalue determined by two-tailedttest unless stated otherwise. Source data are provided as a Source Data file. 7d, f and Figure S 4d , differential expression was calculated using egdeR (3.24.3). Downstream analysis GSEA was performed using the GSEA software (3.0) on pre-ranked differential expression lists. Reporting summary Further information on research design is available in the Nature Research Reporting Summary linked to this article.